Large enhancement in neurite outgrowth on a cell membrane-mimicking conducting polymer Although electrically stimulated neurite outgrowth on bioelectronic devices is a promising means of nerve regeneration, immunogenic scar formation can insulate electrodes from targeted cells and tissues, thereby reducing the lifetime of the device. Ideally, an electrode material capable of electrically interfacing with neurons selectively and efficiently would be integrated without being recognized by the immune system and minimize its response. Here we develop a cell membrane-mimicking conducting polymer possessing several attractive features. This polymer displays high resistance towards nonspecific enzyme/cell binding and recognizes targeted cells specifically to allow intimate electrical communication over long periods of time. Its low electrical impedance relays electrical signals efficiently. This material is capable to integrate biochemical and electrical stimulation to promote neural cellular behaviour. Neurite outgrowth is enhanced greatly on this new conducting polymer; in addition, electrically stimulated secretion of proteins from primary Schwann cells can also occur on it. Bioelectronic devices for nerve regeneration and neuroprosthesis are advancing towards electrically interfacing with tissues with high selectivity, long-term stability and spatial resolution [1] , [2] , with the ultimate goal of stimulating and guiding neurite outgrowth efficiently within very short periods of time. Progress is currently reaching a bottleneck, however, because traditional electronic materials, mostly metals and inorganic semiconductors, cannot satisfy the requirements of matching mechanical strength with biological systems [3] , [4] , high biocompatibility [5] , [6] , and stable electrical transduction [7] , [8] , [9] , [10] , [11] that are necessary for interfacial communication between materials and neural cells. Therefore, the focus has shifted recently towards the application of electrically conducting polymers (ECPs), which are conductors (or semiconductors) like metals, but with the ability to readily tailor their structures through covalent modification of their organic frameworks. Because ECPs have mechanical properties comparable with those of the extracellular matrix (ECM), they should be more compatible with neural cells and tissues than inorganic materials [12] , [13] . ECPs can conduct both electrons and ions, thereby facilitating effective electron—ion transitions over device–tissue boundaries with low impedance [14] , [15] , [16] , [17] . Pioneering studies have demonstrated the efficiency of using ECPs for electrical interfacing with neural cells and tissues [18] , [19] , [20] , [21] , [22] , [23] , [24] , [25] , [26] . Langer and coworkers [24] first demonstrated a 90% enhancement in the length of neurite outgrowth after electrical stimulation on unfunctionalized polypyrrole. Subsequently, various means of integrating ECPs and biofunctional groups, through physical mixing or chemical immobilization, have been tested [27] , [28] , [29] , [30] . For example, Schmidt and coworkers [27] coated electrospun poly(lactic- co -glycolic acid) nanofibres with polypyrrole and applied this material for neural engineering. Separately, the same group also immobilized nerve growth factor onto the surface of polypyrroles with the application of an adhesion layer for similar purpose [29] . Wallace and coworkers [31] employed a different approach to form polypyrrole/collagen complexes stabilized through electrostatic interactions. Unfortunately, these modifications usually lead to relatively lower degrees of enhancement in neurite outgrowth, presumably because of the lower conductivity of these materials [29] . Recent research interests on ECP-based devices shift the focus to polyethylenedioxythiophenes (PEDOTs) [25] , [26] . PEDOTs display stability in aqueous solution when a voltage is applied, a critical feature for medical devices implanted for long periods of time [14] , [15] , [16] , [18] , [32] . In addition, the interfacial impedance of PEDOT at 1 kHz is not only significantly less than that of Pt [33] but also smaller than that of iridium oxide [10] , one of the most investigated electrode materials. PEDOT also displays a large charge storage capability with a small potential excursion [10] , [11] . These outstanding electrical properties allow PEDOT to provide stable electrical communications with attached cells and tissues, and efficiently deliver charges to them over extended periods of time [34] . PEDOTs have already been employed to interface with neural tissues and cells in many bioelectronic devices [35] , including electronic ion pumps for neural signal delivery [36] , transistors for biosensing [37] , [38] , cochlear implants [39] and neural probes [40] . An implanted bioelectronic device would, ideally, establish stable and long-term electrical communication with living tissues, thereby allowing regeneration of the tissues or an exchange of physiological signals to recover damaged biofunctions. Unfortunately, most commercially available ECPs, including unfunctionalized PEDOTs, are likely to encounter implant-induced inflammation, even though the conditions after implantation may not be as severe as those resulting from implantation of metals and inorganic semiconductors [15] , [41] , [42] . If these ECPs cannot discriminate among proteins and cells, proteins, microphages and astrocytes might also accumulate on the surface of the polymers. This phenomenon would initialize the inflammatory response and scar formation, thereby insulating the electrodes from the targeted cells and tissues and causing the device to lose its ability to function [43] , [44] . To resolve this issue, several groups have focused on tuning the biological and physical functions of ECPs through chemical modification or dopant switching. For example, Povlich et al . [45] conjugated RGD peptide onto PEDOT chemically and observed that the new polymer could induce neural differentiation. Although the introduction of oligopeptide ligands (for example, YIGSR [46] , RGD), collagen [31] , or nerve growth factor [21] can enhance cell—material interactions, thereby stabilizing cell proliferation and differentiation, no corresponding decreases in immunogenic response have been observed [43] , [46] . When Wadhwa et al. [47] doped anti-inflammatory drugs and neurotrophic factors into polymer films to enhance the biocompatibility of ECPs, they had limited success, controlling inflammation for only short periods of time. This approach might not be promising for long-term implantation because the drug would eventually be consumed [19] , [43] . Here, we show the design and synthesis of ethylenedioxythiophene (EDOT)—based polymers that specifically recognize neural cells, thereby endowing neural bioelectronics with the inherent capability to resist nonspecific binding of proteins and cells and, as a result, allowing electrical communication with cells over extended periods of time. We follow a cell membrane-mimicking approach to synthesize biomimetic PEDOTs consisting of two new EDOT monomers. Taking a cue from the structure of phospholipids, we prepare a phosphorylcholine-grafted EDOT to resist nonspecific binding to both proteins and cells; we also develop a maleimide-grafted EDOT for conjugation with peptide ligands to mimic specific integrin—ECM interactions. These biomimetic PEDOTs are not only inert in normal biological environments but also interact specifically with target cells after covalent linking with peptide ligands. Moreover, this biomimetic design imparts the materials with low electrical impedance [48] , [49] , thereby allowing intimate and stable electrical communication between the materials and the cells/tissues over long periods of time. Utilizing this material, we observe the respective and integrated effects of biochemical and electrical stimulations for neural cell engineering and record large enhancement of neurite outgrowth and protein secretion on neural cells. Design and synthesis of biomimetic PEDOTs To construct an ideal conducting polymer interface, we adopted an approach mimicking the inertness and specific binding properties of cell membranes ( Fig. 1a ), which mainly comprise phospholipid bi-layers with imbedded proteins, carbohydrates and other biopolymers to direct surface functions [50] . The outer layer is predominated by the polar zwitterionic phosphorylcholine heads of phospholipids; the great hydrophilicity of these zwitterionic interfaces creates the inertness and nonthrombogenic properties [51] , [52] , [53] . Moreover, specific binding between cells and the ECM is mediated by membrane integrins and ECM peptide segments, with the subsequent anchoring of cells onto the ECM promoting tissue formation. To integrate these features, we prepared two new EDOT monomers ( Fig. 1b ). Starting from hydroxymethyl-functionalized EDOT (EDOT-OH), we introduced a zwitterionic phosphorylcholine functional group, simulating a phospholipid, onto EDOT (giving the new monomer EDOT-PC), using a procedure similar to those reported previously for the preparation of phosphorylcholine-functionalized polyacrylates and self-assembled monolayers [54] , [55] , [56] , [57] . EDOT-OH was first reacted with 2-chloro-2-oxo-1,3,2-dioxaphospholane (COP); the dioxaphospholane ring was subsequently opened in the presence of trimethylamine to yield the phosphorylcholine functional group. The non-crystalline product was purified through normal-phase column chromatography with a high-polarity solvent (a combination of EtOAc, MeOH, water and MeCN). Under the optimized reaction and purification conditions, we could synthesize EDOT-PC in quantities greater than 10 g. We also synthesized a maleimide-functionalized EDOT (EDOT-MI) for covalent conjugation to the integrin-recognized peptide sequence [58] . 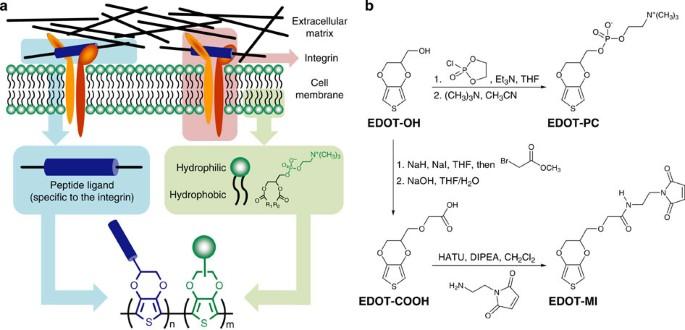Figure 1: Design and synthesis of the biomimetic conducting polymer. (a) Schematic representation of the approach leading to the design of the target conducting polymer, mimicking the interactions between a cell membrane and the ECM. (b) Syntheses of new EDOT-based monomers designed through the biomimetic approach. Figure 1: Design and synthesis of the biomimetic conducting polymer. ( a ) Schematic representation of the approach leading to the design of the target conducting polymer, mimicking the interactions between a cell membrane and the ECM. ( b ) Syntheses of new EDOT-based monomers designed through the biomimetic approach. Full size image Electropolymerization from a mixture of functionalized EDOT monomers directly onto electrode surfaces allowed the rapid formation of multifunctional conducting polymers. We found, however, that hydrophilic EDOT-PC could not be electrodeposited onto electrodes from aqueous electrolyte solutions; in addition, this monomer was almost insoluble in the organic solvents commonly used for electrochemistry. Moreover, the opposing polarities of EDOT-PC and EDOT-MI made it challenging to find a co-solvent system for electropolymerization of these two monomers at different feed compositions. To overcome these challenges, we developed a protocol for electropolymerization using the surfactant dioctyl sodium sulphosuccinate (DSS). In the presence of DSS, EDOT-PC dissolved in MeCN without the need to introduce a secondary solvent, presumably because of strong ionic interactions between the zwitterionic phosphorylcholine head and the anionic surfactant. On applying a cyclic potential between −0.6 and +1.0 V, we could polymerize and deposit the dissolved EDOT-PC onto various electrode substrates, including indium tin oxide (ITO), gold and stainless steel ( Supplementary Fig. 1 ). Using atomic force microscopy, we estimated the thickness of the polymer film prepared from a single scan to be 20 nm, increasing with each subsequent scan. Interfacial behaviours The prepared poly(EDOT-PC) films exhibited water droplet contact angles of less than 8°. They displayed excellent resistance towards nonspecific binding of proteins, including bovine serum albumin, fibronectin, fibrinogen, lysozyme, and fetal bovine serum, as revealed in Fig. 2a . In contrast, poly(EDOT-OH) films bound strongly to proteins. We also examined the binding of PC12 cells to these polymers. The poly(EDOT-PC) films exhibited no adhesion ( Fig. 2b ); their resistance towards the adhesion of both proteins and cells most likely resulted from the highly hydrophilic yet net-neutral properties of the zwitterionic groups on their surfaces [59] . The poly(EDOT-PC) films retained their good cell resistance after exposure for 30 days to a medium containing 10% horse serum and 10% FBS, suggesting that films deposited from the monomer EDOT-PC would be promising for long-term recording applications. 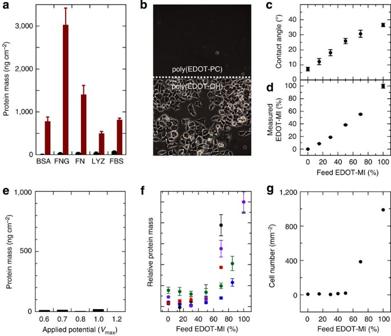Figure 2: Characterization and interfacial properties of biomimetic PEDOTs. (a) Absorption of various proteins (bovine serum albumin, fibronectin (FN), fibrinogen (FNG), lysozyme (LYZ), FBS) on poly(EDOT-PC) (black) and poly(EDOT-OH) (red). (b) Micrograph image of PC12 cells selectively attached and cultured on functionalized poly(EDOT) films for 24 h. Poly(EDOT-PC) was selectively deposited onto the upper part of poly(EDOT-OH). (c–f) Characterization and surface properties of poly(EDOT-MI-co-EDOT-PC)s prepared with different EDOT-MI feed compositions: (c) contact angles of water droplets; (d) measured compositions of EDOT-MI determined through X-ray photoelectron spectroscopy; (e) enzyme resistance tests of poly(EDOT-PC) after the polymer had been subjected to the applied potential for 1,000 cycles in aqueous solution (legends on thexaxis indicate the maximum applied potential); (f) absorption of BSA (black), FN (blue), FNG (red), LYZ (green) and FBS (purple) (the absorbed protein mass relative to the value obtained from pure poly(EDOT-MI) is used as theyaxis so that the absorption trends of different proteins can be compared); (g) density of PC12 cells attached to poly(EDOT-MI-co-EDOT-PC)s prepared with different feed compositions. The error bars in the graphs represent s.d. from at least three repeating experiments. Figure 2: Characterization and interfacial properties of biomimetic PEDOTs. ( a ) Absorption of various proteins (bovine serum albumin, fibronectin (FN), fibrinogen (FNG), lysozyme (LYZ), FBS) on poly(EDOT-PC) (black) and poly(EDOT-OH) (red). ( b ) Micrograph image of PC12 cells selectively attached and cultured on functionalized poly(EDOT) films for 24 h. Poly(EDOT-PC) was selectively deposited onto the upper part of poly(EDOT-OH). ( c – f ) Characterization and surface properties of poly(EDOT-MI- co -EDOT-PC)s prepared with different EDOT-MI feed compositions: ( c ) contact angles of water droplets; ( d ) measured compositions of EDOT-MI determined through X-ray photoelectron spectroscopy; ( e ) enzyme resistance tests of poly(EDOT-PC) after the polymer had been subjected to the applied potential for 1,000 cycles in aqueous solution (legends on the x axis indicate the maximum applied potential); ( f ) absorption of BSA (black), FN (blue), FNG (red), LYZ (green) and FBS (purple) (the absorbed protein mass relative to the value obtained from pure poly(EDOT-MI) is used as the y axis so that the absorption trends of different proteins can be compared); ( g ) density of PC12 cells attached to poly(EDOT-MI- co -EDOT-PC)s prepared with different feed compositions. The error bars in the graphs represent s.d. from at least three repeating experiments. Full size image The surfactant electropolymerization method also allowed us to copolymerize EDOT-PC with EDOT-MI in MeCN. Indeed, we could copolymerize these two immiscible monomers over an entire range of EDOT-MI feed compositions (molar percentage within the monomer mixture) from 0 to 100% ( Supplementary Fig. 1 ). The water contact angles of the poly(EDOT-MI- co -EDOT-PC) films increased almost linearly from 8 to 36.5° on increasing the EDOT-MI feed composition ( Fig. 2c ). X-ray photoelectron spectroscopy revealed that the binding energy of the N 1s electrons of EDOT-PC (396.3 eV) was higher than that of EDOT-MI (393.8 eV). Because the two N 1s signals overlapped, we used a non-linear least squares fitting procedure to accurately calculate the compositions of the copolymer films ( Supplementary Fig. 2 ). As revealed in Fig. 2d , the measured EDOT-MI compositions in the copolymers were slightly lower than the feed EDOT-MI compositions. Nevertheless, the copolymer composition was almost linearly dependent on the monomer feed composition. Although poly(EDOT-PC) was hydrophilic, it was very stable in aqueous buffers, even after applying a potential sweep over 1,000 cycles. The electroactivity of the film decreased slightly, but the protein resistance remained intact, even when the maximum applied potential reached 1.2 V ( Fig. 2e and Supplementary Fig. 3 ). Poly(EDOT-PC) and all copolymer films were smooth and exhibited similar surface roughness (root mean square roughness ( R rms )=ca. 3 nm; Supplementary Fig. 4 ), as determined using atomic force microscopy. Instead of a linear relationship, the surface resistance of the copolymer films towards the binding of cells and proteins exhibited a sigmoidal dependence on the EDOT-MI feed composition ( Fig. 2f,g ). When the feed composition of EDOT-MI in the monomer mixture was less than 50%, the electropolymerized films were highly resistant towards cells and proteins. In contrast, when the EDOT-MI content exceeded 50%, cells and proteins bound strongly to the copolymer films. The phenomenon observed was similar to the studies on zwitterionic group-tailored self-assembled monolayers [54] . Only for the experiments of FBS binding, the maleimide groups on poly(EDOT-MI- co -EDOT-PC)s needed to be blocked by cysteine before the protein resistance test. This was due to the large quantity of free thiol groups on FBS proteins. Therefore, instead of physical absorption, we observed chemical conjugation in quartz crystal microbalance (QCM) experiments without cysteine blocking. Peptide bioconjugation and controlled adhesion of cells The peptide Ile-Lys-Val-Ala-Val (IKVAV) is one of the active sites in laminin for neuron adhesion and neurite outgrowth [60] , [61] . This peptide ligand has been used extensively to support the adhesion and differentiation of neuronal origin cells, including PC12 cells, Granule cells, Purkinje cells, neural progenitor cells and hippocampal neurons. We achieved bioconjugation through reactions between maleimides and cysteine-terminated experimental (CSSSSIKVAV) and control (CSSSSGKVAV) peptides in phosphate buffer at an optimized pH of 5.6; these reactions were complete within an hour, as monitored using an in situ QCM ( Fig. 3a ). In contrast, we detected no bioconjugation in the case of the non-cysteine-capped peptide SSSSIKVAV. The density of ligands grafted on the polymer films could be controlled by varying the composition of the copolymers; it reached ~3,000 ng cm −2 when the feed composition of EDOT-MI was greater than 50% ( Fig. 3b ). PC12 cells are commonly employed as a model system for studies of neuronal development and function; they are also a robust model cell line for evaluating the performance of various platforms for electrically stimulated neurite outgrowth [24] , [27] , [28] , [29] , [30] . To compare the performance of our materials with that of other reported platforms, we also adopted PC12 cells in this study to investigate neuron adhesion and differentiation. The introduction of IKVAV promoted PC12 cell binding on the originally bioinert poly(EDOT-MI- co -EDOT-PC), the result of specific ligand—receptor interactions. The density of attached cells increased rapidly on increasing the content of EDOT-MI to 10%, becoming saturated thereafter ( Fig. 3c ). Control experiments with GKVAV revealed no attachment of PC12 cells. All of the PC12 cells were adhered and well extended on the IKVAV-grafted copolymer films when the feed content of EDOT-MI was greater than 10%. 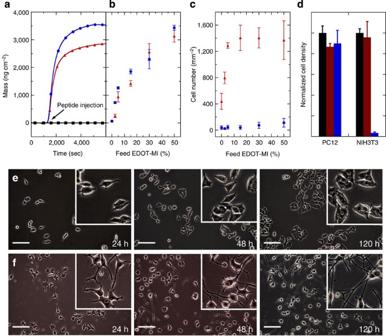Figure 3: Ligand conjugation and controlled cellular behaviour on biomimetic PEDOTs. (a)In situmonitoring of CSSSSIKVAV (red), CSSSSGKVAV (blue) and SSSSIKVAV (black) conjugation on poly(EDOT-MI-co-EDOT-PC) films polymerized from a monomer solution containing 5 mM EDOT-MI and 5 mM EDOT-PC. (b) Conjugation of CSSSSIKVAV (red) and CSSSSGKVAV (blue) on poly(EDOT-MI-co-EDOT-PC) films prepared with various EDOT-MI feed compositions. (c) Density of PC12 cells attached to poly(EDOT-MI-co-EDOT-PC) films, prepared with different feed compositions, after conjugation with the ligands CSSSSIKVAV (red) and CSSSSGKVAV (blue). The error bars in the graphs represent s.d. from at least three repeating experiments. (d) Selective adhesion of PC12 and NIH3T3 cells on a polystyrene culture dish (black), poly(EDOT-OH) (red) and a biomimetic PEDOT (prepared from 3 mM EDOT-MI and 7 mM EDOT-PC, conjugation with IKVAV; blue) after cell seeding for 1 day. (e) Proliferation and (f) differentiation (in the presence of NGF) of PC12 cells attached to CSSSSIKVAV-conjugated poly(EDOT-MI-co-EDOT-PC) films after 24, 48 and 120 h. The insets are enlarged micrograph images of cultured cells to confirm the cellular morphologies. The length of the scale bars in the micrograph images is 200 μm. Figure 3: Ligand conjugation and controlled cellular behaviour on biomimetic PEDOTs. ( a ) In situ monitoring of CSSSSIKVAV (red), CSSSSGKVAV (blue) and SSSSIKVAV (black) conjugation on poly(EDOT-MI- co -EDOT-PC) films polymerized from a monomer solution containing 5 mM EDOT-MI and 5 mM EDOT-PC. ( b ) Conjugation of CSSSSIKVAV (red) and CSSSSGKVAV (blue) on poly(EDOT-MI- co -EDOT-PC) films prepared with various EDOT-MI feed compositions. ( c ) Density of PC12 cells attached to poly(EDOT-MI- co -EDOT-PC) films, prepared with different feed compositions, after conjugation with the ligands CSSSSIKVAV (red) and CSSSSGKVAV (blue). The error bars in the graphs represent s.d. from at least three repeating experiments. ( d ) Selective adhesion of PC12 and NIH3T3 cells on a polystyrene culture dish (black), poly(EDOT-OH) (red) and a biomimetic PEDOT (prepared from 3 mM EDOT-MI and 7 mM EDOT-PC, conjugation with IKVAV; blue) after cell seeding for 1 day. ( e ) Proliferation and ( f ) differentiation (in the presence of NGF) of PC12 cells attached to CSSSSIKVAV-conjugated poly(EDOT-MI- co -EDOT-PC) films after 24, 48 and 120 h. The insets are enlarged micrograph images of cultured cells to confirm the cellular morphologies. The length of the scale bars in the micrograph images is 200 μm. Full size image In earlier studies of ECPs for neural engineering, most research was focused on the performance of unfunctionalized ECP. In vivo applications of these materials may suffer, however, from the unwanted nonspecific binding of cells and biomacromolecules, leading to severe insulating scar formation and failure of electrical communication with living tissues. Previous investigations of non-conductive materials have concluded that the presence of phosphorylcholine side chains can prevent microphages from recognizing artificial implants as foreign bodies, leading to diminution/eradication of the inflammatory response [55] . We expected the biomimetic PEDOTs developed herein to interact specifically with targeted cells and prevent nonspecific binding. A standard cell culture dish and poly(EDOT-OH) revealed strong adhesion to both PC12 cells and NIH3T3 fibroblasts ( Fig. 3d ). In contrast, the biomimetic PEDOT films presenting IKVAV ligands remained resistant to NIH3T3 cells ( Supplementary Fig. 6 ), binding only to the PC12 cells. This behaviour resulted from the two principles we employed in the molecular design: the introduction of phosphorylcholine side chains to prevent nonspecific interactions and the presence of the conjugated IKVAV ligand for specific interactions with PC12 cells, but not with NIH3T3 fibroblasts. To the best of our knowledge, this paper is the first to demonstrate neuron-targeting conducting polymers that function without nonspecific interactions—a highly attractive feature for in vivo applications because of the low host inflammatory response towards the conducting polymers and the greater long-term performance of related materials and devices after implantation. After the cells had attached to the surface of biomimetic PEDOTs, they proliferated in the presence of serum proteins ( Fig. 3e ), with the polymers sustaining culturing for more than 20 days. The cell viability and proliferation were similar to those when cultured on polylysine-coated dishes. PC12 cells also underwent normal differentiation in the presence of nerve growth factor ( Fig. 3f ). In control experiments performed using unfunctionalized PEDOT films, most of the cells did not spread well and were presented in smaller, circular shapes. The results were even worse on the poly(EDOT-OH) films. One major concern after chemical modification of ECPs is decreased conductivity because of distortion of their backbones, thereby diminishing orbital overlap and weakening intrachain conductivity. The introduction of insulating side chains to improve the solubility can also lead to the presence of insulating domains in bulk materials, again resulting in poor interchain conductivity. Accordingly, the electrical impedance would increase and the electrical communication would worsen. We suspected, however, that the introduction of a zwitterionic phosphorylcholine unit onto the EDOT monomer would not only interrupt the nonspecific interactions but also maintain the impedance of the PEDOT materials for electron/ion injection, due to its higher ionic conductivity [48] , [49] . As revealed in Supplementary Fig. 5 , the impedance of poly(EDOT-MI- co -EDOT-PC) was even lower than that of the unfunctionalized PEDOT film, and almost one order of magnitude lower than that of a gold film in the low frequency range. In general, the impedance could also be affected by the surface morphology of electrodes because the rougher surface with larger surface area allowed higher rate of charge injections. Therefore, rougher surfaces would result in lower impedance. As shown in Supplementary Fig. 4 , both unfunctionalized PEDOT and poly(EDOT-MI- co -EDOT-PC) films displayed surface R rms of less than 10 nm. Actually, the PEDOT film showed larger R rms than the poly(EDOT-MI- co -EDOT-PC) film. However, its impedance was higher, thereby excluding the difference of surface area as the main factor for the low impedance of poly(EDOT-MI- co -EDOT-PC) film. After the conjugation of insulating peptide (IKVAV) on poly(EDOT-MI- co -EDOT-PC), the impedance raised slightly but was still comparable to that of PEDOT. This low impedance of biomimetic PEDOT would ensure efficient delivery or recording of electrical signals. Integration of biochemical and electrical stimulations The most attractive feature of ECP-based materials over traditional polymer- or biopolymer-based materials is their ability to allow electrical stimulation of adhered cells and tissues. Conventional ECPs are, however, unlikely to possess the stability and biocompatibility required to sustain long-term electrical stimulation for tissue regeneration and function recovery after implantation. As a result of their designed ligand—receptor interactions and decreased nonspecific physical absorption of cells, we suspected that the biological and electrical stability of our biomimetic PEDOTs would be much greater than those of PEDOTs that rely on physical absorption, doping or affinity binding [18] . We employed a home-designed cell culturing device to apply electrical stimulation during the culturing of the cells ( Fig. 4a ). We electrodeposited the biomimetic PEDOT films onto an ITO-coated glass substrate featuring an insulating gap between the fabricated pairs of transparent electrodes. After the PC12 cells had been seeded onto the substrate under conditions to differentiate, we applied a biphasic electrical pulse ( Fig. 4b ) to the electrodes to stimulate the cells. 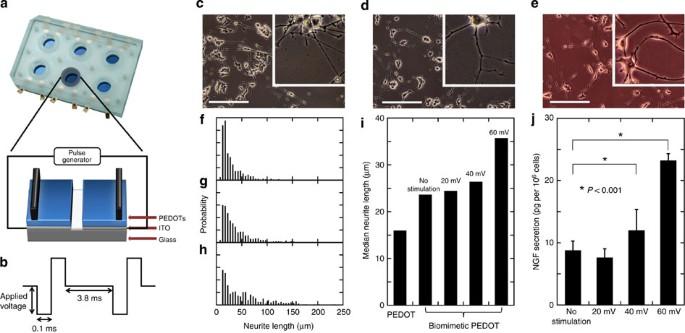Figure 4: Electrically stimulated cell behaviour on biomimetic PEDOTs. (a) Schematic representation of the device used for cell growth with applied electrical stimulation. (b) Illustration of the electrical pulse used. (c–e) Microscopy images of differentiated PC12 cells cultured in NGF-supplemented medium for 5 days on (c) a PEDOT film, (d) a biomimetic PEDOT film (prepared from 3 mM EDOT-MI and 7 mM EDOT-PC, conjugation with IKVAV), and (e) the biomimetic PEDOT film with applied pulsed electrical stimulation at an amplitude of 60 mV. The insets are enlarged micrograph images of cultured cells to confirm the cellular morphologies. The length of the scale bars in the micrograph images is 200 μm. (f–h) Corresponding neurite length distributions of (c–e). (i) Median neurite length of PC12 cells on PEDOT and biomimetic PEDOT in the absence and presence of applied pulsed electrical stimulation at amplitudes of 20, 40 and 60 mV. (j) NGF secretion from primary Schwann cells cultured on biomimetic PEDOTs (prepared from 3 mM EDOT-MI and 7 mM EDOT-PC, conjugation with RGD) in the absence and presence of applied pulsed electrical stimulation at amplitudes of 20, 40 and 60 mV. Figure 4: Electrically stimulated cell behaviour on biomimetic PEDOTs. ( a ) Schematic representation of the device used for cell growth with applied electrical stimulation. ( b ) Illustration of the electrical pulse used. ( c – e ) Microscopy images of differentiated PC12 cells cultured in NGF-supplemented medium for 5 days on ( c ) a PEDOT film, ( d ) a biomimetic PEDOT film (prepared from 3 mM EDOT-MI and 7 mM EDOT-PC, conjugation with IKVAV), and ( e ) the biomimetic PEDOT film with applied pulsed electrical stimulation at an amplitude of 60 mV. The insets are enlarged micrograph images of cultured cells to confirm the cellular morphologies. The length of the scale bars in the micrograph images is 200 μm. ( f – h ) Corresponding neurite length distributions of ( c – e ). ( i ) Median neurite length of PC12 cells on PEDOT and biomimetic PEDOT in the absence and presence of applied pulsed electrical stimulation at amplitudes of 20, 40 and 60 mV. ( j ) NGF secretion from primary Schwann cells cultured on biomimetic PEDOTs (prepared from 3 mM EDOT-MI and 7 mM EDOT-PC, conjugation with RGD) in the absence and presence of applied pulsed electrical stimulation at amplitudes of 20, 40 and 60 mV. Full size image Our first observation was that neurite outgrowth of PC12 cells was greatly promoted on the biomimetic PEDOTs. Because the neurite length displayed non-Gaussian distribution, following the previous studies [24] , [31] , we used median neurite length as the numerical indicator to evaluate and compare the experimental results. In a control experiment performed on PEDOT ( Fig. 4c ), the PC12 cells possessed a median neurite length of 15.9 μm after being differentiated in the presence of nerve growth factor for 5 days ( Fig. 4f,i ); some of these cells were not well spread and had a more circular shape. Moreover, the condition of the cells was even worse on the poly(EDOT-OH) films. Compared with the cells differentiated on PEDOT, Fig. 4d reveals that the PC12 cells adhered and spread much better on the biomimetic PEDOT [IKVAV-conjugated poly(EDOT-MI- co -EDOT-PC)]; the median neurite length increased from 48% to 23.3 μm under the same conditions ( cf . Fig. 4g,i ). The presence of the IKVAV moieties not only ensured specific attachment of the PC12 cells but also stimulated the neurite outgrowth [60] , [61] . Greater than 99% of the PC12 cells remained viable after we had applied pulsed electrical stimulation at an amplitude of 60 mV for 8 h per day and 5 days in a row ( Fig. 4e ). This stimulation time was significantly longer than those reported from most previously conducted cell-based electrical stimulation experiments [20] , [24] , [27] , [28] , [29] , [30] . In contrast, greater than 40% of the cells detached from unfunctionalized PEDOTs after only 1 day of electrical stimulation at an even lower voltage (20 mV). We observed substantial increases in neurite outgrowth on the biomimetic PEDOTs when the peak voltage was set at 20, 40 or 60 mV ( Fig. 4i ). The median neurite length was greatest at 60 mV, without any effect on cell viability. After we had stimulated the PC12 cells for 5 days, it was clearly observed that more longer neurites were formed. After electrical stimulation, the median neurite length reached 35.7 μm, corresponding to a 124% enhancement of original value (15.9 μm) on PEDOT (cf. Fig. 4h,i ). Comparison of cumulative distribution plots of neurite length ( Supplementary Fig. 7 ) also revealed similar conclusion because greater number of long neurites were presented. This increase is significantly greater than not only the values (20–60%) typically reported on hybrid and functionalized conducting organic materials [20] , [27] , [28] , [29] , [30] but also the largest increase (90%) previously reported on polypyrrole [24] . We attribute this behaviour to the integrated stimulation of surface biochemical ligands and applied electrical pulses. To demonstrate that our approach of preparing biomimetic PEDOT could also be applied to other cells as an integrated platform for biochemical and electrical stimulation, we turned our focus to primary Schwann cells (glial cells that function to support neurons in the peripheral nervous system). These cells play a key role in nerve regeneration by secreting neurotrophic factors that help the axon sprouts grow towards the injured neurons [62] . Several reports demonstrated that the secretion/expression of both brain-derived neurotrophic factor and neuron growth factor (NGF) were elevated on electrical stimulation [63] , [64] , [65] . Similar to the situation described above, our poly(EDOT-MI- co -EDOT-PC) films were inert towards the Schwann cells in the absence of attached ligands. On conjugation of the peptide GRGDSP, however, the Schwann cells adhered specifically to the films. We monitored the secretion of NGF in the absence of electrical stimulation and in the presence of the same electrical pulses as described above (that is, amplitudes of 20, 40 and 60 mV). Figure 4j reveals that NGF secretion from the Schwann cells was enhanced after electrical stimulation at amplitudes of 40 and 60 mV, relative to that from the control experiment performed without electrical stimulation. When applying a pulse having a peak voltage of 60 mV, the NGF secretion reached a level of 23.19 pg per 10 6 cells—an enhancement of 165% when compared with the original NGF secretion without stimulation (8.77 pg per 10 6 cells). When integrating biochemical and electrical stimulation, such biomimetic PEDOTs might allow rapid nerve regeneration after device implantation. In a search for materials that would allow bioelectronic devices to interface with nerve cells and provide stable, efficient and long-term electrical communication, we have developed membrane-biomimicking conducting polymers based on EDOT. We synthesized these new polymer films from a pair of monomers: a zwitterionic phosphorylcholine-functionalized EDOT (EDOT-PC) and a maleimide-functionalized EDOT (EDOT-MI). These films are easy to fabricate through a unique surfactant-assisted polymerization; their compositions can be tuned simply by varying the ratio of monomers in the initial mixture. These biomimicking PEDOTs display high electrical/ionic conductivities, enabling efficient electrical communication at cell—material interfaces. They also exhibit high resistance towards the nonspecific binding of enzymes and cells, allowing them to be functional in aqueous buffers for extended periods of time and promising to diminish immunogenic responses. In addition, selective binding of desired cells can be achieved to ensure intimate electrical interfacing through specific ligand—receptor interactions (we demonstrate herein a unique example of a specific neuron-targeting conducting polymer). Finally, the biomimetic PEDOTs display low impedance in the low frequency range, ideal for biological applications. The combination of these features enables two desirable material characteristics. The first is stable binding and electrical communication between the biomimetic PEDOTs and their attached neural cells. As a result, these cells can be electrically stimulated for 8 h a day for 5 days in a row without any observed cell detachment and death. We suspect that electrical stimulation can be extended even further. The second characteristic is that the ligands presented on the surface also provide biochemical stimulation to allow differentiation of the attached cells. Accordingly, this material integrates both biochemical and electrical stimulation. Taking advantage of all of these attractive features, we achieved a 124% enhancement—significantly greater than the 20–90% enhancements previously reported—in the median neurite length of differentiated PC12 cells on electrical stimulation on the ECPs. Moreover, we have demonstrated enhanced NGF secretion by 165% from primary Schwann cells on similar electrical stimulation. If these biomimetic PEDOT materials were to be integrated with implanted bioelectronic devices, these features would ensure intimate electrical communication with targeted nerve tissues and efficient delivery of electrical signals, thereby enabling long-term electrical interfacing with tissues. The application of this approach towards biomimetic conducting copolymers is not be limited merely to the field of neural interfacing; it can be extended further through specifically targeted ligand—receptor interactions and cell—electronics interfaces. The features of these polymers are critical and desired for in vivo applications of bioelectronic devices. The stability and device–tissue electrical communication will be ensured by preventing severe immunogenic responses and formation of insulating scars. Together with our collaborating researchers, we are now investigating the promising applications of these materials for nerve regeneration and in neuroprosthetic devices and biosensors. Synthesis of materials and measurements EDOT-OH was purchased from a custom-synthesis company, where it had been prepared following procedures previously reported [66] , [67] . EDOT-COOH was synthesized following procedures previously reported [68] , [69] . 2-Maleimidoethylamine hydrochloride and 1-ethyl-3-(3-dimethyaminopropyl)-carbodiimide hydrochloride were purchased from Astatech and Tokyo Chemical Industry, respectively. The photoresist (50–60% TCIR-ZR9000PB in propylene glycol monomethyl ether acetate) and developer (2.38% tetramethylammonium hydroxide in H 2 O) were purchased from Tokyo Ohka Kogyo and Tama Chemicals, respectively. All materials for cell culturing were purchased from Invitrogen. All other chemicals were purchased either from Sigma-Aldrich or Wako Pure Chemical Industries. CH 2 Cl 2 and tetrahydrofuran were dried and purified using a PureSolv MD 5 Solvent Purification System (Innovative Technology); all other chemicals were of reagent grade and used as received. 1 H and 13 C NMR spectra were recorded at 25 °C using a Varian 500 NMR spectrometer operated at 500 and 125 MHz, respectively; chemical shifts are reported relative to tetramethylsilane; the signal of the residual non-deuterated solvent was taken as the secondary reference. EDOT-PC COP (1.65 g, 11.6 mmol) was added slowly to a solution of EDOT-OH (2.00 g, 11.6 mmol) in dry tetrahydrofuran (30 ml) and triethylamine (20 ml) at −29 °C while stirring under a N 2 atmosphere. After maintaining the temperature at −20 to −30 °C for 3 h, the mixture was heated slowly to 25 °C and then stirred for further 3 h. The precipitate (triethylamine hydrochloride) was filtered off and then the filtrate was concentrated in vacuo to provide (2-chloro-2-oxo-1,3,2-dioxaphospholoyloxy)-3,4-EDOT (EDOT-COP), quantitatively, as light yellow liquid. Trimethylamine (2.67 g, 4.52 mmol) was added rapidly to a solution of EDOT-COP (3.14 g, 11.3 mmol) in MeCN (10 ml) in a 100 ml pressure vessel at −29 °C. After sealing, the pressure vessel was heated at 60 °C for 16 h. The formation of product was monitored by thin layer chromatography and observed by ultraviolet/visible light (365 nm wavelength). The product's retardation factor was 0.14 using a mixed solvent of EtOAc/MeOH/H 2 O/MeCN (3/1/1/1). The flask was cooled back to −29 °C, causing a light yellow viscous liquid to precipitate. This precipitate was filtered off and purified chromatographically (SiO 2 ; EtOAc/MeOH/H 2 O/MeCN) to give the yellow solid 1 (3.30 g, 9.78 mmol, 84.3% isolated yield). 1 H NMR (500 MHz, D 2 O): 6.51 (s, 2 H), 4.46–4.43 (m, 1 H), 4.31–4.24 (m, 3 H), 4.16–4.06 (m, 3 H), 3.65–3.56 (m, 2 H), 3.19 (s, 9 H) p.p.m. 13 C NMR (125 MHz, D 2 O): 140.55, 140.38, 100.46, 72.74, 65.94, 65.30, 63.70, 59.41, 53.92 p.p.m. High resolution mass spectrometry (FAB) [M+H] + calcd for [C 12 H 20 O 6 NPS+H] + : m / z 338.0827; found 338.0844. EDOT-MI 2-Maleimidoethylamine hydrochloride (0.42 g, 2.39 mmol) and N , N -diisopropylethylamine (0.49 ml, 2.39 mmol) were added sequentially to a solution of EDOT-COOH (0.500 g, 2.17 mmol) and O -(7-azabenzotriazol-1-yl)- N , N , Ń , Ń -tetramethyluronium hexafluorophosphate (0.91 g, 2.39 mmol) in dry dimethylformamide (15 ml) under an N 2 atmosphere at 0 °C. The formation of product was monitored by thin layer chromatography and observed by ultraviolt/visible light (365 nm wavelength). The product's retardation factor was 0.33 using a mixed solvent of EtOAc/hexane (2/1). After stirring for 6 h at room temperature, the mixture was diluted with EtOAc (100 ml), washed with brine (3 × 100 ml), dried (MgSO 4 ), filtered and concentrated under reduced pressure. Chromatographic purification (SiO 2 ; EtOAc/hexane gradient) afforded the white solid 2 (0.72 g, 2.04 mmol, 85% isolated yield). 1 H NMR (500 MHz, DMSO- d 6 ): 7.87 (t, J =6.0 Hz, 1 H), 6.97 (s, 2 H), 6.57 (s, 2 H), 4.35–4.31 (m, 1 H), 4.27 (dd, J =11.5, 2.0 Hz, 1 H), 4.02 (dd, J =11.5, 7.5 Hz, 1 H), 3.83 (s, 2 H), 3.65–3.58 (m, 2 H), 3.48 (t, J =8.3 Hz, 2 H), 3.23 (q, J =6.1 Hz, 2 H) p.p.m. 13 C NMR (125 Hz, DMSO- d 6 ): 171.51, 169.60, 141.76, 141.70, 134.93, 100.19, 100.17, 72.67, 70.68, 69.61, 65.78, 40.46, 40.30, 40.13, 39.96, 39.80, 39.63, 39.46, 37.47, 37.20 p.p.m. High resolution mass spectrometry (FAB) [M+H] + calcd for [C 15 H 17 N 2 O 6 S+H] + : m / z 353.08073; found 353.08189. Electropolymerization of EDOT and electrochemical analysis Electrochemical experiments were performed using an Autolab PGSTAT128N potentiostat (Metrohm Autolab) and a three-electrode electrochemical cell, with a Pt electrode as the counter electrode and an Ag/AgNO 3 electrode (0.01 M AgNO 3 and 0.1 M Bu 4 NPF 6 in MeCN) as the reference electrode. Each measurement was calibrated using a standard ferrocene/ferrocenium redox system. EDOT-PC is highly hydrophilic, but could be dissolved in organic electrolytes with the aid of the surfactant DSS. EDOT-PC could be electropolymerized onto conducting substrates as thin films under electrooxidation. If not stated otherwise, EDOT derivatives were electropolymerized or copolymerized on conducting substrates from 0.01 M solutions in MeCN containing 0.05 M DSS and 0.1 M LiClO 4 on applying cyclic potential scans. Electrochemical impedance spectroscopy (EIS) was performed using a sinusoidal excitation signal with an excitation amplitude of 10 mV at 50 frequencies logarithmically spaced from 10 kHz to 1 Hz. The conducting polymer films for measurements were coated on fresh Au substrates (area: 1 cm 2 ). Before recording EIS spectra, samples were conditioned in PBS buffer at 0.23 V for 60 s. EIS was registered at 25 °C in the PBS buffer with 10 mM [Fe(CN) 6 ] 3−/4− (1:1, mol/mol) as the redox couple. QCM measurements QCM-D measurements were performed at 25 °C on a Q-Sense AB system (Biolin Scientific) to monitor in situ the interactions of biomolecules with the functionalized conducting polymer substrates. The conducting polymers were electrochemically deposited on the surface of a QSX 301 sensor crystal (Biolin Scientific) and then placed in the measurement chamber. Solutions of the biomolecules were delivered continuously to the measurement chamber at a flow rate of 20 μl min −1 , pumping with an Ismatec ISM597D pump. On interaction of the matter in solution with the substrate on the sensor crystal, the changes in the resonance frequency of the sensor (Δ f ), which is related to the attached mass, were recorded at a resolution of less than 1 s. If necessary, the pump was stopped for a few seconds to change the sample solutions without disturbing the QCM-D signal. The resonance frequencies were measured simultaneously at 5 MHz and its five harmonics (15, 25, 35, 45, 55 and 65 MHz). If not stated otherwise, changes in frequency of the third overtone ( n =3; that is, 15 MHz) are presented. Cell culture with in vitro electrical stimulation Rat pheochromocytoma (PC12) and NIH3T3 cells were obtained from the RIKEN Cell Bank. Primary rat Schwann cells were purchased from ScienCell Research Laboratories. Following typical procedures for cell differentiation, PC12 cells were seeded at a density of 1 × 10 4 /cm 2 onto EDOT polymer thin films deposited on ITO glass substrates assembled in a homemade culture chamber ( Fig. 4a ) and then incubated for 12 h to permit attachment and spreading before initiating electrical stimulation. The ITO substrate was separate into two equal parts by a 400-μm insulating linear gap (fabricated through confined acid etching). Charge-balanced biphasic electrical stimulation at 250 Hz ( Fig. 4b ) was produced using a B2912A precision source/measure unit (Agilent); two parts of the EDOT polymer-coated ITO substrates served as electrodes to release electrical signals to the cells. The major advantage of the biphasic electrical stimulation was that it could maintain charge balance while minimizing cell damage. After the initial 12 h of incubation, the PC12 cells were subjected to electrical stimulation for more than 5 days (8 h per day). The amplitude of the biphasic pulse was 20, 40 or 60 mV. The differentiation results for PC12 cells subjected to a 100-mV pulse for 5 days are not included because the viability of the PC12 cells was highly decreased in this case. PC12 cells plated on the same PEDOT thin films, but not subjected to any electrical stimulation, served as controls; cells grown on unfunctionalized EDOT polymer thin films, but not subjected to any electrical stimulus, served as additional controls. The morphological features of all cells were examined every 24 h. Primary rat Schwann cells were seeded at a density of 5 × 10 3 cm −2 on the polymer substrates. The settings, programs and parameters for their electrical stimulation were the same as those adopted for the PC12 cells. The Schwann cells were cultured for 72 h and then they were subjected to the electrical pulse for more than 3 days (8 h every day). Schwann cells plated on the same PEDOT thin films, but not subjected to any electrical stimulation, served as controls. The culture medium was refreshed every 24 h. After 3 days of electrical stimulation, the culture medium was accumulated for detection of NGF. Detection of NGF secretion Secretion of NGF by the Schwann cells was determined using a two-site ELISA assay (NGF E max Immunoassay System, Promega). Experiments were performed as instructed by the technical bulletin, using the supernatant of the Schwann cells. The absorbance of each sample after colour development was measured using a Wallac Victor 1420 Multilabel Counter (PerkinElmer). A one-way analysis of variance was used to assess statistical differences between NGF samples secreted under different conditions. How to cite this article : Zhu, B. et al. Large enhancement in neurite outgrowth on a cell membrane-mimicking conducting polymer. Nat. Commun. 5:4523 doi: 10.1038/ncomms5523 (2014).